DrosophilaStrip serves as a platform for early endosome organization during axon elongation Early endosomes are essential for regulating cell signalling and controlling the amount of cell surface molecules during neuronal morphogenesis. Early endosomes undergo retrograde transport (clustering) before their homotypic fusion. Small GTPase Rab5 is known to promote early endosomal fusion, but the mechanism linking the transport/clustering with Rab5 activity is unclear. Here we show that Drosophila Strip is a key regulator for neuronal morphogenesis. Strip knockdown disturbs the early endosome clustering, and Rab5-positive early endosomes become smaller and scattered. Strip genetically and biochemically interacts with both Glued (the regulator of dynein-dependent transport) and Sprint (the guanine nucleotide exchange factor for Rab5), suggesting that Strip is a molecular linker between retrograde transport and Rab5 activation. Overexpression of an active form of Rab5 in strip -mutant neurons suppresses the axon elongation defects. Thus, Strip acts as a molecular platform for the early endosome organization that has important roles in neuronal morphogenesis. Neurons are highly polarized cells, possessing two morphologically and functionally distinct domains, axons and dendrites [1] , [2] . In developing neurons, membrane trafficking is essential for delivering diverse organelles and molecules that are required for elongation and guidance of the growing axon or dendrite processes [3] , [4] , [5] . Especially bi-directional endosomal trafficking between cell body and neurite termini is crucial to respond to continuously changing surrounding environments; endosomal trafficking regulates the number and activity of cell surface molecules at the neurite termini in time and space [6] . For example, brain-derived neurotrophic factor (BDNF)-driven Trk receptor endocytosis at growth cone affects axon growth [7] , [8] . Asymmetric clathrin-mediated endocytosis of adhesion receptors such as integrins is required for repulsive growth cone guidance [9] . Among vesicular structures in the endocytic pathway, early endosomes are essential for cell signalling, serving both as signalling centres and as sorting centres to degrade or recycle cargoes [10] , [11] . The organization of early endosomes consists of three steps; endocytosis, clustering and fusion. Internalized small early endosomes are clustered and then undergo fusion to become matured early endosomes. Rab5 is a key regulator for ligand sequestration at the plasma membrane and repetitive fusion of internalized early endosomes by recruiting its effectors such as VPS34/p150, EEA1, Rabaptin-5 and Rabenosyn-5 (Rbsn-5) (refs 12 , 13 , 14 , 15 , 16 , 17 ). In addition, the dynein-dependent transport of small early endosomes from the periphery to the cell centre is important for clustering them [18] , [19] . Recently, the essential roles of endocytosis in axon elongation of mouse sympathetic neurons [7] and endocytosis and endosomal trafficking in the dendrite arborization of Drosophila dendritic arborization (da) sensory neurons [20] , [21] were reported. However, the physiological significance of clustering of early endosomes and the molecular link between the transport/clustering and Rab5 activity are largely unknown. We here performed a forward genetic mosaic screen to identify genes for their cell autonomous functions in dendrite and axonal development, and identified an evolutionarily conserved protein, Striatin-interacting protein (Strip), that works as a molecular linker between retrograde transport and Rab5 activity in early endosome organization. Strip and its orthologues were reported to be a component of Striatin-interacting phosphatase and kinase (STRIPAK) complex [22] , [23] , [24] ; however, the function of Strip has not been reported yet, to our knowledge. Interestingly, we found that Strip forms the protein complex with both Glued, the orthologue of mammalian p150 Glued , and Sprint, the orthologue of RIN-1. Glued is an essential component of the dynactin complex and regulates the initiation of retrograde transport on microtubule [25] , [26] , [27] , [28] , [29] , and Sprint is supposed to be a guanine nucleotide exchange factor (GEF) for Rab5 (refs 30 , 31 ). We found that Strip affects the transport of early endosomes by forming complex with Glued in developing neurons. Furthermore, clustering of early endosomes is defective in strip -knockdown Drosophila S2 cells and HeLa cells; early endosomes become smaller and scattered as reported in dynein-inhibited HeLa cells [18] . Moreover, similar to other GEFs, Sprint and Strip have a higher affinity for guanosine diphosphate (GDP)-bound forms of Rab5 than for guanosine triphosphate (GTP)-bound form. In addition, Strip seems to stabilize protein level of Sprint. Finally, the expression of constitutively active form of Rab5 in strip -mutant neurons suppresses the axon elongation defect. These data demonstrate that Strip coordinates dynein-dependent transport and Rab5 activation at the clustering and fusion of early endosomes, which are required for axon elongation. strip dogi PNs show defects in neuronal morphogenesis Drosophila olfactory projection neurons (PNs) ( Fig. 1a ), which are analogous to vertebrate mitral/tufted cells, provide an excellent model system for studying the molecular mechanisms of neuronal morphogenesis. Neuronal targeting and branching patterns of PNs are genetically defined [32] , [33] , [34] , and the mosaic analysis with a repressible cell marker (MARCM) method allows us to manipulate the genotype of a single PN (single-cell clone) or of a group of PNs that share the same lineage (neuroblast clone) and are positively labelled in vivo [35] . We performed a MARCM-based forward genetic screen of PNs to identify the genes essential for neuronal morphogenesis [36] , and isolated a mutant doubled glomeruli ( dogi ). As we will mention below, the causal gene of dogi mutant is strip gene; thus, we name this mutant allele strip dogi hereafter. Wild-type PN axons target two higher olfactory centres, the mushroom body and the lateral horn, whereas dendrites target specific glomeruli in the antennal lobe, the first olfactory centre consisting of ~50 glomeruli [32] , [37] , [38] ( Fig. 1a,b ). In neuroblast clones homozygous for strip dogi , neuronal guidance and targeting were severely defective, including ectopic innervation to the contralateral antennal lobe ( Fig. 1d , dotted circle) or the subesophageal ganglion (SOG) ( Fig. 1d , arrowhead), which was never observed in wild-type neuroblast clones ( Fig. 1c ). 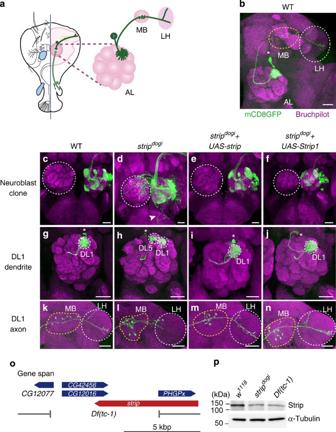Figure 1: Branching and elongation defects ofstripdogihomozygous projection neurons. Schematic view of projection neurons (PNs). Olfactory information is transmitted from the olfactory receptor neurons (light green) to PNs (dark green) at the antennal lobe (AL, pink circle). The dendrite of a single PN targets a specific glomerulus out of 50 glomeruli in the AL, while the axon elongates and branches at the mushroom body (MB) and the lateral horn (LH). (b) Representative image of wild-type (WT) DL1 mosaic analysis with a repressible cell marker (MARCM) clone, DL1 PN (green). Magenta: Bruchpilot staining. Asterisk: cell body. Yellow and white dotted circles indicate MB and the LH, respectively. (c–f) Representative images of WT (c),stripdogineuroblast clones (d),stripdogineuroblast clones expressing cDNA ofstrip(e) or cDNA of mouse homolog ofstrip,Strip1(f). Contralateral ALs are marked by dotted circles, and neurite innervation to suboesophageal ganglion (SOG) is indicated by an arrowhead (d). (g–n) Representative images of DL1 MARCM single-cell clone of each genotype. (g–j) Dendrites of DL1 PNs. DL1 and DL5 glomeruli are indicated by dotted circles, and cell bodies are labelled with asterisks. (k–n) Axons of DL1 PNs. Yellow and white dotted circles indicate the mushroom body (MB) and the lateral horn (LH), respectively. Scale bar: 25 μm. (o) Genomic structure ofstrip. The small deletion alleleDf(tc-1)lacks 7 kb of the genomic region containingstrip, CG42456, CG12016 and CG12077. Scale bar: 5 kbp. (p) Strip expression in WT, the zygotic mutant homozygous forstripdogiorDf(tc-1). Embryo lysates from 18–21 h after egg-laying (AEL) were used for immunoblotting; Strip protein was detected by the anti-Strip antibody. The Strip protein is about 130 kDa. Figure 1: Branching and elongation defects of strip dogi homozygous projection neurons. Schematic view of projection neurons (PNs). Olfactory information is transmitted from the olfactory receptor neurons (light green) to PNs (dark green) at the antennal lobe (AL, pink circle). The dendrite of a single PN targets a specific glomerulus out of 50 glomeruli in the AL, while the axon elongates and branches at the mushroom body (MB) and the lateral horn (LH). ( b ) Representative image of wild-type (WT) DL1 mosaic analysis with a repressible cell marker (MARCM) clone, DL1 PN (green). Magenta: Bruchpilot staining. Asterisk: cell body. Yellow and white dotted circles indicate MB and the LH, respectively. ( c – f ) Representative images of WT ( c ), strip dogi neuroblast clones ( d ), strip dogi neuroblast clones expressing cDNA of strip ( e ) or cDNA of mouse homolog of strip , Strip1 ( f ). Contralateral ALs are marked by dotted circles, and neurite innervation to suboesophageal ganglion (SOG) is indicated by an arrowhead ( d ). ( g – n ) Representative images of DL1 MARCM single-cell clone of each genotype. ( g – j ) Dendrites of DL1 PNs. DL1 and DL5 glomeruli are indicated by dotted circles, and cell bodies are labelled with asterisks. ( k – n ) Axons of DL1 PNs. Yellow and white dotted circles indicate the mushroom body (MB) and the lateral horn (LH), respectively. Scale bar: 25 μm. ( o ) Genomic structure of strip . The small deletion allele Df(tc-1) lacks 7 kb of the genomic region containing strip, CG42456, CG12016 and CG12077 . Scale bar: 5 kbp. ( p ) Strip expression in WT, the zygotic mutant homozygous for strip dogi or Df(tc-1) . Embryo lysates from 18–21 h after egg-laying (AEL) were used for immunoblotting; Strip protein was detected by the anti-Strip antibody. The Strip protein is about 130 kDa. Full size image To examine PN morphologies at a higher resolution, we generated single-cell clones homozygous for strip dogi (hereafter we call this single neuron as strip dogi PN). PNs that target a single glomerulus are categorized into ~50 classes, each with stereotyped dendrite and axon branching patterns [32] , [37] , [38] . In the wild-type DL1 PN, dendrites targeted the posterior, dorsolateral glomerulus DL1 and arborized within the DL1 glomerulus ( Fig. 1b,g ), whereas the axon exhibited stereotypical L-shape branching in the lateral horn ( Fig. 1b,k ). In the strip dogi DL1 PN, both axons and dendrites were defective. Unlike wild-type PNs, in which the dendrite shaft is generated by one branch that forms off the main branch and never branches further, strip dogi PN dendrites had an additional branch appearing from the proximal side of the dendrite shaft (magnified image in Fig. 2f arrowhead, penetrance of additional branch: 35.3%, n =24/68), resulting in dendrite targeting of two glomeruli rather than a single glomerulus ( Fig. 1h ). The axons of strip dogi DL1 PNs did not elongate or form L-shaped branches within the lateral horn ( Fig. 1l , penetrance of short axon: 98.2%, n =56/57). 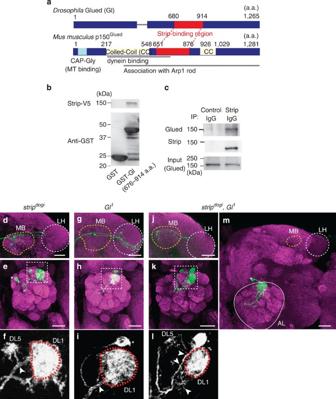Figure 2: Glued (Gl) physically and genetically interacts with Strip. (a) Comparison betweenDrosophilaGl and its mouse orthologue, p150Glued. The 680–914 amino-acid region of Gl bound strongly to Strip in a yeast two-hybrid screen. This is analogous to the 651–876 amino-acid region of p150Glued(68.9% similarity and 23.0% identity); this region interacts with the dynein motor protein and the Arp1 rod. (b) Lysates of 0–22 h after egg-laying (AEL) embryos that express Strip-V5 were pulled down with GST-fused Gl domain that binds to Strip in the yeast two-hybrid screen. (c) Immunoprecipitation of S2 lysates. Endogenous Gl was co-immunoprecipitated when endogenous Strip was precipitated by the anti-Strip antibody. (d–m) Genetic interactions betweenstripandGlin projection neurons (PNs). MARCM DL1 single-cell clones forstripdogi(d–f),Gl1(g–i), or bothstripdogiandGl1(j–m) were generated at 0–24 h ALH (green). Magenta: Bruchpilot staining. Scale bar: 25 μm. (d,g,j) Axons. Yellow and white dotted circles indicate the mushroom body (MB) and the lateral horn (LH), respectively. (e,f,h,i,k,l) Dendrites. Cell bodies are indicated by asterisks. (f), (i), and (l) are magnified images of dotted rectangles of (e), (h), and (k), respectively. Only green channels are shown in grey scale. DL1 glomeruli are labelled with dotted red circles. Additional dendrite branches are indicated by arrowheads. (m) Representative image ofstripdogiandGl1DL1 PN exhibiting the ‘extremely short axon’ phenotype; the axon did not exit the antennal lobe (AL, white circle) and did not enter the mushroom body (MB, yellow dotted circle) or the lateral horn (LH, white dotted circle). Figure 2: Glued (Gl) physically and genetically interacts with Strip. ( a ) Comparison between Drosophila Gl and its mouse orthologue, p150 Glued . The 680–914 amino-acid region of Gl bound strongly to Strip in a yeast two-hybrid screen. This is analogous to the 651–876 amino-acid region of p150 Glued (68.9% similarity and 23.0% identity); this region interacts with the dynein motor protein and the Arp1 rod. ( b ) Lysates of 0–22 h after egg-laying (AEL) embryos that express Strip-V5 were pulled down with GST-fused Gl domain that binds to Strip in the yeast two-hybrid screen. ( c ) Immunoprecipitation of S2 lysates. Endogenous Gl was co-immunoprecipitated when endogenous Strip was precipitated by the anti-Strip antibody. ( d – m ) Genetic interactions between strip and Gl in projection neurons (PNs). MARCM DL1 single-cell clones for strip dogi ( d – f ), Gl 1 ( g – i ), or both strip dogi and Gl 1 ( j – m ) were generated at 0–24 h ALH (green). Magenta: Bruchpilot staining. Scale bar: 25 μm. ( d , g , j ) Axons. Yellow and white dotted circles indicate the mushroom body (MB) and the lateral horn (LH), respectively. ( e , f , h , i , k , l ) Dendrites. Cell bodies are indicated by asterisks. ( f ), ( i ), and ( l ) are magnified images of dotted rectangles of ( e ), ( h ), and ( k ), respectively. Only green channels are shown in grey scale. DL1 glomeruli are labelled with dotted red circles. Additional dendrite branches are indicated by arrowheads. ( m ) Representative image of strip dogi and Gl 1 DL1 PN exhibiting the ‘extremely short axon’ phenotype; the axon did not exit the antennal lobe (AL, white circle) and did not enter the mushroom body (MB, yellow dotted circle) or the lateral horn (LH, white dotted circle). Full size image Strip is required for PN morphogenesis To identify the causal gene for these strip dogi PN phenotypes, we performed meiotic recombination mapping using single-nucleotide polymorphisms (SNPs) [39] and P-elements [40] ; this placed the strip dogi mutation in an ~28-kb region of 63D1 (see Methods for details). Within this region, we generated a small deletion allele, Df(tc-1 ), which lacked 7 kb of the genomic region containing strip ( CG11526 ), CG42456, CG12016 and CG12077 ( Fig. 1o ). The MARCM Df(tc-1) clones exhibited defects in axon elongation, similar to those seen in strip dogi PNs ( Supplementary Fig. 1a ), and also in dendrite branching ( Supplementary Fig. 1b,c arrowheads), which was observed in some strip dogi PNs ( Fig. 2e,f arrowhead). Next, we generated a short-hairpin RNA against strip ( shRNA-strip ) to knock down strip expression; the expression of shRNA-strip in wild-type DL1 PN recapitulated the dendrite branching and axon elongation defects seen in strip dogi PNs ( Supplementary Fig. 1d–f ; see Supplementary Fig. 1g–j for the evaluation of shRNA - strip ). Lastly, the expression of strip cDNA in strip dogi PN clones rescued all the strip dogi phenotypes ( Fig. 1e,i,m ). These findings confirmed that strip is responsible for the strip dogi PN phenotypes and is cell autonomously required for neuronal morphogenesis, specifically for dendrite branching and axon elongation. Strip protein is highly conserved from yeast to humans ( Supplementary Fig. 1k ), with 45.9% amino-acid identity and 81.4% similarity between Drosophila and human STRIP1, and known as a component of Striatin-interacting phosphatase and kinase (STRIPAK) complex [22] , [23] , [24] . However, Strip has no characterized functional domains and its function has not been studied yet. When the mouse orthologue of strip , Strip1 (refs 41 , 42 ) (MGI: 2443884) was expressed only in strip dogi PNs using the MARCM strategy, all the strip dogi phenotypes were rescued ( Fig. 1f,j,n ), suggesting that the function of Strip is conserved between Drosophila and mammals. To characterize the Strip protein, we generated an antibody against Strip and confirmed its reliability by staining PNs homozygous for Df(tc-1) at 0 h after puparium formation (APF) ( Supplementary Fig. 1l–o ); immunostaining was not observed in Df(tc1) -homozygous cell bodies ( Supplementary Fig. 1o ). This result indicates that Strip is expressed in PNs during dendrite branching and axon elongation. Then, we used the Strip antibody for western blotting of embryo lysates from zygotic strip dogi and Df(tc-1) mutants, and found that the amount of Strip protein was significantly and similarly reduced in both lysates ( Fig. 1p ). The remaining expression of Strip in zygotic strip dogi or Df(tc-1) mutants is probably due to the maternally derived strip gene product. Thus, the strip dogi allele used for phenotypic analysis is a strong loss-of-function or null allele. Strip interacts with Glued and Sprint To examine how Strip regulates dendrite branching and axon elongation, we performed a yeast two-hybrid screen using full-length Strip as bait and the Drosophila whole-embryo cDNA library as prey, and identified Glued (Gl) and Sprint (Spri) as the binding partners of Strip ( Figs 2a and 3a ). Gl is a major component of the dynactin complex, which is a positive regulator of the microtubule (MT)-dependent retrograde motor, dynein, and regulates the initiation of retrograde transport [25] , [26] , [27] , [28] , [29] . Gl and its mouse orthologue, p150 Glued , have an MT-binding domain, a dynein intermediate chain-binding domain and an Arp1-associated domain ( Fig. 2a ). The Gl cDNA fragment isolated from the yeast two-hybrid screen encoded 235 amino acids, from position 680 to 914, corresponding to the dynein- or Arp1-binding domain ( Fig. 2a ). We confirmed this physical interaction by performing glutathione S -transferase (GST) pull-down and co-immunoprecipitation using Drosophila embryos and Drosophila S2 cell lysates ( Fig. 2b,c ). The other binding partner of Strip, Spri, is an orthologue of human RIN-1 and has a vacuolar protein sorting 9 (VPS9) domain that is crucial for its function as a GEF for the small GTPase protein, Rab5 (ref. 43 ) ( Fig. 3a ). The spri cDNA fragment isolated from the yeast two-hybrid screen encoded 397 amino acids, from position 1,404 to 1,700, corresponding to the VPS9 domain ( Fig. 3a ). We also confirmed this interaction by performing GST pull-down and co-immunoprecipitation using Drosophila embryos and Drosophila S2 cell lysates ( Fig. 3b–d ). 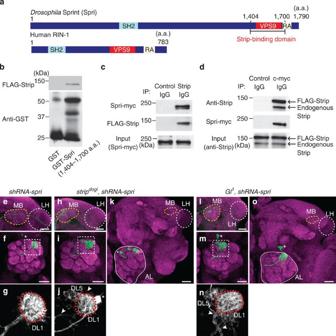Figure 3: Sprint (Spri) physically and genetically interacts with Strip. (a) Comparison betweenDrosophilaSpri and its human orthologue, RIN-1. The 1,404–1,700 amino-acid region of Spri bound strongly to Strip in a yeast two-hybrid screen. This is analogous to the vacuolar protein sorting homology domain 9 (VPS9) that is required for guanine nucleotide exchange activity. SH2: Src homology domain 2, RA: Ras association domain. (b) Lysates of 0–22 h after egg-laying (AEL) embryos expressing FLAG-tagged Strip (FLAG-Strip) was pulled down with GST-fused Spri (Strip binding domain). (c,d) Immunoprecipitation of S2 lysates expressing c-myc tagged Spri (Spri-myc) and FLAG-Strip. Spri-myc was co-immunoprecipitated when FLAG-Strip was precipitated by the anti-Strip antibody (c). FLAG-Strip was co-immunoprecipitated when Spri-myc was precipitated by the anti-c-myc antibody. Since FLAG-Strip was detected with the anti-Strip antibody, the lower band represents endogenous Strip (d). (e–o) Genetic interactions betweenspriandstrip or spri and Glin projection neurons (PNs). MARCM DL1 single-cell clones expressingshRNA-spri(e–g),stripdogiDL1 single-cell clones expressingshRNA-spri(h–k), orGl1DL1 single-cell clones expressingshRNA-spri(l–o) were induced (green) at 0–24 h ALH. Magenta: Bruchpilot staining. Scale bar: 25 μm. (e,h,l) Axons. Yellow and white dotted circles indicate the mushroom body (MB) and the lateral horn (LH), respectively. (f,g,i,j,m,n) Dendrites. Cell bodies are indicated by asterisks. (g), (j), and (n) are magnified images of dotted rectangles of (f), (i), and (m), respectively. Only green channels are shown in grey scale. DL1 glomeruli are labelled with dotted red circles. Additional dendrite branches are indicated by arrowheads. (k,o) Representative images ofstripdogiDL1 PNs expressing theshRNA-spri(k), andGl1DL1 PNs expressing theshRNA-spri(o) exhibiting the ‘extremely short axon’ phenotype, i.e., the axon did not exit the antennal lobe (white circle) and did not enter the mushroom body (MB, yellow dotted circle) or the lateral horn (LH, white dotted circle). Figure 3: Sprint (Spri) physically and genetically interacts with Strip. ( a ) Comparison between Drosophila Spri and its human orthologue, RIN-1. The 1,404–1,700 amino-acid region of Spri bound strongly to Strip in a yeast two-hybrid screen. This is analogous to the vacuolar protein sorting homology domain 9 (VPS9) that is required for guanine nucleotide exchange activity. SH2: Src homology domain 2, RA: Ras association domain. ( b ) Lysates of 0–22 h after egg-laying (AEL) embryos expressing FLAG-tagged Strip (FLAG-Strip) was pulled down with GST-fused Spri (Strip binding domain). ( c , d ) Immunoprecipitation of S2 lysates expressing c-myc tagged Spri (Spri-myc) and FLAG-Strip. Spri-myc was co-immunoprecipitated when FLAG-Strip was precipitated by the anti-Strip antibody ( c ). FLAG-Strip was co-immunoprecipitated when Spri-myc was precipitated by the anti-c-myc antibody. Since FLAG-Strip was detected with the anti-Strip antibody, the lower band represents endogenous Strip ( d ). ( e – o ) Genetic interactions between spri and strip or spri and Gl in projection neurons (PNs). MARCM DL1 single-cell clones expressing shRNA-spri ( e – g ), strip dogi DL1 single-cell clones expressing shRNA-spri ( h – k ), or Gl 1 DL1 single-cell clones expressing shRNA-spri ( l – o ) were induced (green) at 0–24 h ALH. Magenta: Bruchpilot staining. Scale bar: 25 μm. ( e , h , l ) Axons. Yellow and white dotted circles indicate the mushroom body (MB) and the lateral horn (LH), respectively. ( f , g , i , j , m , n ) Dendrites. Cell bodies are indicated by asterisks. ( g ), ( j ), and ( n ) are magnified images of dotted rectangles of ( f ), ( i ), and ( m ), respectively. Only green channels are shown in grey scale. DL1 glomeruli are labelled with dotted red circles. Additional dendrite branches are indicated by arrowheads. ( k , o ) Representative images of strip dogi DL1 PNs expressing the shRNA-spri ( k ), and Gl 1 DL1 PNs expressing the shRNA-spri ( o ) exhibiting the ‘extremely short axon’ phenotype, i.e., the axon did not exit the antennal lobe (white circle) and did not enter the mushroom body (MB, yellow dotted circle) or the lateral horn (LH, white dotted circle). Full size image We next examined the genetic interactions between strip , Gl and spri . Gl 1 (dominant negative form of Gl ) DL1 PNs ( Fig. 2g–i ) or PNs expressing the shRNA-spri ( Fig. 3e–g ) did not exhibit obvious defects in axon elongation ( Figs 2g and 3e ) or dendrite branching ( Fig. 2h,i arrowhead, 3f,g). Interestingly, axon elongation or dendrite branching phenotypes of strip dogi DL1 PNs ( Fig. 2d–f ) became more severe by adding Gl 1 (double mutant clones for strip dogi and Gl 1 , Fig. 2j–m ) or expressing the shRNA-spri ( Fig. 3h–k ). In both cases, we observed an extremely short axon phenotype, that is, the axon did not exit the antennal lobe ( Fig. 2m (penetrance of extremely short axon: 15.6%, n =5/32) and 3k (penetrance of extremely short axon: 13.0%, n =3/23)), which was never observed in strip dogi DL1 PNs (penetrance of extremely short axon: 0%, n =0 /68). We also found an obvious genetic interaction between strip and Gl in the rough-eye phenotype, in which Gl is known to be involved [44] ( Supplementary Fig. 2a–d ). These biochemical and genetic data suggest that Strip functions with Gl and Spri in dendrite branching and axon elongation. As strip dogi , Gl 1 PNs (double mutant clones) and strip dogi PNs expressing shRNA-spri exhibit the similar ‘extremely short axon’ phenotype, we wondered whether Gl and spri genetically interact. As we expected, axon elongation and dendrite branching defects were observed in Gl 1 PNs expressing shRNA-spri ( Fig. 3l–o , penetrance of extremely short axon in o: 38.9%, n =7/18), suggesting that strip , Gl and spri cooperatively regulate axon elongation and dendrite branching. Strip is involved in transporting early endosomes As the main function of Gl is to regulate the initiation of dynein-based retrograde transport [28] , [29] , it is possible that strip dogi mutation affects intracellular transport. Thus, to examine the function of Strip, we first analysed the subcellular localization of synaptotagmin, a representative axonal transport cargo regulated by the dynein-dynactin complex [45] . We expressed haemagglutinin (HA)-tagged synaptotagmin (syt-HA) [46] in single-cell DL1 PN clones. Most of the syt-HA was delivered properly to the presynaptic sites in strip dogi PNs, but some of it accumulated abnormally in the axon stalks ( Supplementary Fig. 2h–j , quantification in k). This accumulation was not observed in wild-type PNs ( Supplementary Fig. 2e–g , quantification in k); thus, abnormal accumulation of syt-HA in strip dogi PN axon did not result from syt-HA overexpression. These data indicate that Strip is required for the intracellular transport of synaptic proteins in PN axons. We also found defective subcellular localization of early endosomes in strip dogi PNs. As the proper regulation of endosomal trafficking is required for neuronal morphogenesis [6] , we hypothesized that Strip affects the transport of early endosomes during axon elongation. When the early endosome marker, the green florescent protein (GFP)-fused FYVE domain (GFP-FYVE) [47] , was expressed in developing wild-type PNs, it was mainly localized at the termini but not in the stalk of axons at 21 h after puparium formation ( Fig. 4a–c , quantification in g). Interestingly, GFP-FYVE showed significantly higher levels in the axon stalk of strip dogi PNs ( Fig. 4d–f , quantification in g) compared with that in the control ( Fig. 4a–c , quantification in g). Thus, Strip affects the subcellular localization of early endosomes in PN axons when axon elongation is taking place. 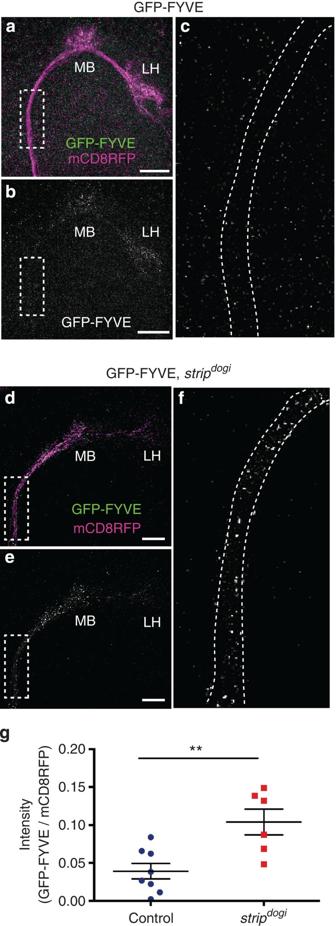Figure 4: Localization of early endosomes was altered in the axons of developingstripprojection neurons (PNs). (a–f) A GFP-fused FYVE domain (GFP-FYVE) was expressed in PNs, and its localization was investigated at 21 h after puparium formation (APF). Axons of wild-type (WT,a–c) andstripdogiPNs (d–f). (a,d) GFP-FYVE and MARCM neuroblast clones labelled by mCD8-RFP are shown in green and magenta, respectively. (b,e) Only green channels are shown in grey scale. (c) and (f) are magnified images of dotted rectangles of (b) and (e), respectively. Scale bar: 25 μm. (g) The intensity of GFP-FYVE in the axon stalk (200 μm2) was normalized to the intensity of mCD8RFP and then plotted. Error bars are defined as s.e.m. **P=0.0047,t-test. Figure 4: Localization of early endosomes was altered in the axons of developing strip projection neurons (PNs). ( a – f ) A GFP-fused FYVE domain (GFP-FYVE) was expressed in PNs, and its localization was investigated at 21 h after puparium formation (APF). Axons of wild-type (WT, a – c ) and strip dogi PNs ( d – f ). ( a , d ) GFP-FYVE and MARCM neuroblast clones labelled by mCD8-RFP are shown in green and magenta, respectively. ( b , e ) Only green channels are shown in grey scale. ( c ) and ( f ) are magnified images of dotted rectangles of ( b ) and ( e ), respectively. Scale bar: 25 μm. ( g ) The intensity of GFP-FYVE in the axon stalk (200 μm 2 ) was normalized to the intensity of mCD8RFP and then plotted. Error bars are defined as s.e.m. ** P =0.0047, t -test. Full size image Strip and Gl are involved in clustering of early endosomes To examine the effect of Strip on endosomal trafficking, the localization of Rab5- and Avalanche (Avl; Drosophila orthologue of Syntaxin 7, 12) [48] -positive early endosomes was examined in Drosophila S2 cells. The organization of early endosomes consists of three steps; endocytosis, clustering and fusion ( Fig. 5a ). Retrograde transport is required for clustering of internalized vesicles (small early endosomes) that are formed by endocytosis [18] , [19] . After clustering, small early endosomes undergo homotypic fusion to form mature early endosomes [12] , [13] , [15] . Interestingly, the size of Rab5- and Avl-positive early endosomes was significantly affected in S2 cells treated with strip dsRNA. Enlarged Rab5- and Avl-positive early endosomes were frequent in cells treated with control dsRNA ( Fig. 5b,e , Rab5 is quantified in Fig. 5h, and Avl is quantified in Fig. 5i), but they were smaller in cells treated with strip dsRNA ( Fig. 5c,f,h,i ). Next, we tried to elucidate which step of the early endosome organization is defective in strip knockdown. We examined the endocytosis ability of cells treated with strip dsRNA using the FM1-43 styryl dye and found that strip knockdown did not inhibit endocytosis ( Supplementary Fig. 3 , see Methods for details). Furthermore, the same ‘smaller Rab5- and Avl-positive early endosomes’ phenotype was observed when the cells were treated with Gl dsRNA ( Fig. 5d,g–i ). These results suggest that Strip affects, at least, the clustering of early endosomes by forming a complex with Gl, which is consistent with the previous report that dynein-dependent early endosome transport from the periphery to the centre of a cell is required for the organization of early endosomes [18] , [19] . We also revealed that Strip function in early endosome clustering is evolutionarily conserved. We treated HeLa cells with control or human STRIP1 siRNA and stimulated them with fluorescent-labelled-EGF (EGF-Alexa488) for 3 min followed by washing to remove labelled EGF from the medium ( Fig. 6a ). Like FM1-43 dye uptake assay performed in Drosophila S2 cells, endocytosis of EGFR bound to EGF-Alexa488 was not defective in STRIP1 siRNA-treated HeLa cells, suggesting that STRIP1 knockdown does not inhibit endocytosis. EGF-Alexa488-positive vesicles were localized at cell periphery both in control or STRIP1 siRNA-treated HeLa cells just after washing out the EGF-Alexa488 ( Fig. 6b,c ). After 30 min incubation, the localization of EGF-Alexa488 was different between control and STRIP1 siRNA-treated HeLa cells ( Fig. 6d–g , Supplementary Fig. 4 ). In control cells, EGF-Alexa488-positive vesicles disappeared from cell periphery and mainly localized at peri-nuclear region ( Fig. 6d,e , quantified in Fig. 6h). In contrast, in STRIP1 siRNA-treated HeLa cells, most of the cells possessed small and scattered EGF-Alexa488-positive vesicles, which are mainly at cell periphery ( Fig. 6f,g , quantified in Fig. 6h). In addition, those small EGF-Alexa488-positive vesicles are EEA1 negative ( Supplementary Fig. 4d–f arrowheads), suggesting they are immature early endosomes. Thus, we concluded that Drosophila strip and human STRIP1 are involved in clustering of early endosome organization. 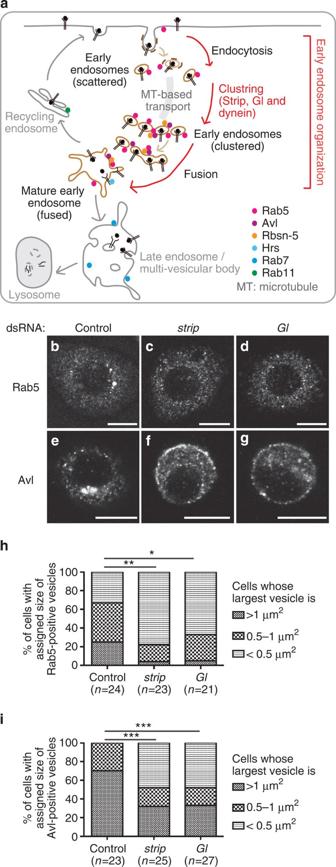Figure 5: Localization defects of early endosomes instripknockdownDrosophilaS2 cells. (a) Schematic view of endocytic pathways. Early endosome organization consists of three steps, endocytosis, clustering and fusion of small early endosomes. (b–g) Localization of early endosome markers (Rab5 and Avalanche, Avl) in the control (b,e),strip(c,f), andGl(d,g) dsRNA-treated S2 cells. (b–d) Rab5-positive early endosomes. (e–g) Avl-positive early endosomes. Scale bar: 7.5 μm. (h,i) Quantification of the size of Rab5-positive early endosomes (h) and Avl-positive early endosomes (i). The area of each vesicle was measured with the Particle Analyzer of the ImageJ software. The percentage of cells whose largest vesicle with sizes >1 μm2, >0.5 μm2but <1 μm2, and <0.5 μm2are shown. *P=0.049, **P=0.0068, ***P<0.0001, chi-square test. Figure 5: Localization defects of early endosomes in strip knockdown Drosophila S2 cells. ( a ) Schematic view of endocytic pathways. Early endosome organization consists of three steps, endocytosis, clustering and fusion of small early endosomes. ( b – g ) Localization of early endosome markers (Rab5 and Avalanche, Avl) in the control ( b , e ), strip ( c , f ), and Gl ( d , g ) dsRNA-treated S2 cells. ( b – d ) Rab5-positive early endosomes. ( e – g ) Avl-positive early endosomes. Scale bar: 7.5 μm. ( h , i ) Quantification of the size of Rab5-positive early endosomes ( h ) and Avl-positive early endosomes ( i ). The area of each vesicle was measured with the Particle Analyzer of the ImageJ software. The percentage of cells whose largest vesicle with sizes >1 μm 2 , >0.5 μm 2 but <1 μm 2 , and <0.5 μm 2 are shown. * P =0.049, ** P =0.0068, *** P <0.0001, chi-square test. 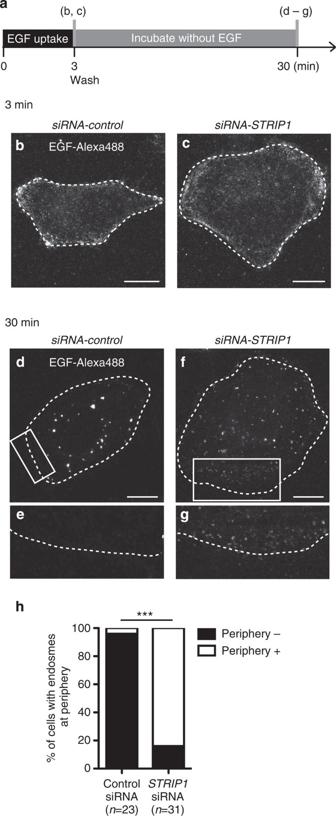Figure 6: Localization defects of EGF-Alexa488 inSTRIP1knockdown HeLa cells. (a) Summary of EGF-Alexa488 uptake assay. (b–g) Localization of EGF-Alexa488 in the control (b,d,e) andSTRIP1(c,f,g) siRNA-treated HeLa cells. HeLa cells were transfected with control orSTRIP1siRNA for 3 days, and endocytosis uptake was assayed with EGF-Alexa488. After a 3 min uptake of EGF-Alexa488, cells were fixed (b,c) or washed with DMEM and cultured for 27 min and fixed (d–g). The rectangle regions of (d) and (f) are magnified at (e) and (g), respectively. Scale bar: 10 μm. (h) All cells were classified into having or not having EGF-Alexa488 at cell periphery by a blind test. ***P<0.0001, chi-square test. Full size image Figure 6: Localization defects of EGF-Alexa488 in STRIP1 knockdown HeLa cells. ( a ) Summary of EGF-Alexa488 uptake assay. ( b – g ) Localization of EGF-Alexa488 in the control ( b , d , e ) and STRIP1 ( c , f , g ) siRNA-treated HeLa cells. HeLa cells were transfected with control or STRIP1 siRNA for 3 days, and endocytosis uptake was assayed with EGF-Alexa488. After a 3 min uptake of EGF-Alexa488, cells were fixed ( b , c ) or washed with DMEM and cultured for 27 min and fixed ( d – g ). The rectangle regions of ( d ) and ( f ) are magnified at ( e ) and ( g ), respectively. Scale bar: 10 μm. ( h ) All cells were classified into having or not having EGF-Alexa488 at cell periphery by a blind test. *** P <0.0001, chi-square test. Full size image Strip regulates axon elongation by controlling Rab5 activity Given that Strip makes complexes with Gl and Spri, we hypothesized that Strip affects the organization of early endosomes by properly clustering them with Gl and promoting early endosome fusion with Spri-Rab5, which are required for axon elongation. To confirm our hypothesis, we first investigated whether Rab5 is required for axon elongation in PNs by generating MARCM single-cell PN clones homozygous for a Rab5 -null mutation [47] ( Fig. 7a ). As in the strip dogi DL1 PN clones, the dendrites in Rab5 2 DL1 PN had additional branches appearing from the proximal side of the dendrite shaft, with a penetrance of 85.7% ( Fig. 7a arrowheads, n =18/21). Some Rab5 2 DL1 dendrites targeted both DL1 and DL5, the same glomeruli targeted by the strip dogi DL1 PNs ( Supplementary Fig. 5 ). In addition, Rab5 2 DL1 PNs had an extremely short axon phenotype (47.6%, n =10/21), that is, the axons stopped in the vicinity of the antennal lobe and did not extend towards the mushroom body or the lateral horn ( Fig. 7a , arrows). These phenotypes were similar to those observed in double mutant clones for strip dogi and Gl 1 ( Fig. 2m ), strip dogi PNs expressing shRNA-spri ( Fig. 3k ) or Gl 1 PNs expressing shRNA-spri ( Fig. 3o ). The expression of yellow fluorescent protein (YFP)-fused Rab5 (YFP-Rab5) [49] rescued Rab5 2 PNs phenotypes ( Fig. 7b,c ), indicating that Rab5 is cell autonomously required for dendrite branching and axon elongation in PNs. 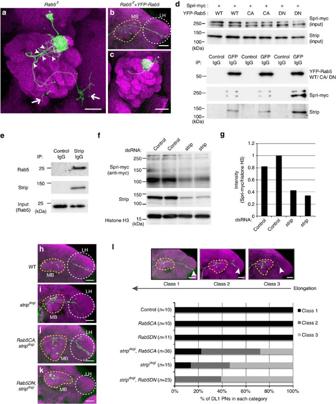Figure 7: Strip affects Rab5 activity in axon elongation. (a–c) Representative image ofRab52DL1 PNs (a, green) andRab52DL1 PNs expressing YFP fused Rab5 (b,c, green). Magenta: Bruchpilot staining. Asterisk: Cell body. Yellow and white dotted circles indicate the mushroom body (MB) and the lateral horn (LH), respectively. Scale bar: 25 μm. (d) Immunoprecipitation of S2 lysates expressing c-myc tagged Spri (Spri-myc) and YFP-tagged Rab5 (YFP-Rab5WT), YFP-tagged dominant negative form of Rab5 (YFP-Rab5DN) or YFP-tagged constitutively active form of Rab5 (YFP-Rab5CA). Spri-myc and Strip were co-immunoprecipitated when YFP-Rab5 WT/CA/DN were precipitated by the anti-GFP antibody. (e) Immunoprecipitation of S2 lysates. The anti-Strip antibody co-immunoprecipitated Strip and endogenous Rab5. (f) The expression level of Spri-myc in control andstripdsRNA-treated S2 cells. Knockdown efficiency was confirmed by anti-Strip antibody and anti-Histone H3 was used as a loading control. (g) Densitometric analysis of Spri-myc in (f). The intensity of Spri-myc was measured by using Image J software and normalized against the intensity of Histone H3 and showed in graph. (h–k) Representative image of DL1 wild-type (WT,h),stripdogiPN (i),stripdogiPN expressing constitutively active form of Rab5 (Rab5CA, Rab5Q88L,j), andstripdogiPN expressing dominant-negative form of Rab5 (Rab5DN, Rab5S43N,k) labelled by mCD8RFP (green). Magenta: Bruchpilot staining. Yellow and white dotted circles indicate the mushroom body (MB) and the lateral horn (LH), respectively. Scale bar: 25 μm. (l) The axons of DL1 PNs were categorized into three classes according to the extent of elongation in a blind test. Class 1 axons reached the end of the LH, while class 3 axons terminated near the mushroom body (l, arrowheads). The percentage of PNs in each category is shown in (l). Figure 7: Strip affects Rab5 activity in axon elongation. ( a – c ) Representative image of Rab5 2 DL1 PNs ( a , green) and Rab5 2 DL1 PNs expressing YFP fused Rab5 ( b , c , green). Magenta: Bruchpilot staining. Asterisk: Cell body. Yellow and white dotted circles indicate the mushroom body (MB) and the lateral horn (LH), respectively. Scale bar: 25 μm. ( d ) Immunoprecipitation of S2 lysates expressing c-myc tagged Spri (Spri-myc) and YFP-tagged Rab5 (YFP-Rab5WT), YFP-tagged dominant negative form of Rab5 (YFP-Rab5DN) or YFP-tagged constitutively active form of Rab5 (YFP-Rab5CA). Spri-myc and Strip were co-immunoprecipitated when YFP-Rab5 WT/CA/DN were precipitated by the anti-GFP antibody. ( e ) Immunoprecipitation of S2 lysates. The anti-Strip antibody co-immunoprecipitated Strip and endogenous Rab5. ( f ) The expression level of Spri-myc in control and strip dsRNA-treated S2 cells. Knockdown efficiency was confirmed by anti-Strip antibody and anti-Histone H3 was used as a loading control. ( g ) Densitometric analysis of Spri-myc in ( f ). The intensity of Spri-myc was measured by using Image J software and normalized against the intensity of Histone H3 and showed in graph. ( h – k ) Representative image of DL1 wild-type (WT, h ), strip dogi PN ( i ), strip dogi PN expressing constitutively active form of Rab5 (Rab5CA, Rab5Q88L, j ), and strip dogi PN expressing dominant-negative form of Rab5 (Rab5DN, Rab5S43N, k ) labelled by mCD8RFP (green). Magenta: Bruchpilot staining. Yellow and white dotted circles indicate the mushroom body (MB) and the lateral horn (LH), respectively. Scale bar: 25 μm. ( l ) The axons of DL1 PNs were categorized into three classes according to the extent of elongation in a blind test. Class 1 axons reached the end of the LH, while class 3 axons terminated near the mushroom body ( l , arrowheads). The percentage of PNs in each category is shown in ( l ). Full size image Next, we examined the physical interactions among Strip, Spri and Rab5. As Spri is an orthologue of RIN-1 that exhibits Rab5-specific guanine nucleotide exchange activity [43] , one would expect that Drosophila Spri could have a higher affinity for GDP-bound forms of Rabs than for GTP-bound forms, which is the common feature of GEFs. As expected, c-myc-tagged Spri (Spri-myc) formed complex preferentially with a dominant negative form of Rab5 (Rab5DN, Rab5S43N) [49] , which mimics the GDP-bound or free form of Rab5, and weakly to constitutively active form (Rab5CA, Rab5Q88L) [49] , which mimics the GTP-bound form ( Fig. 7d ). In accordance with our hypothesis, Strip also had a higher affinity for GDP-bound forms of Rab5 than for GTP-bound forms ( Fig. 7d ). In addition, we also confirmed the physical interaction between endogenous Strip and Rab5 ( Fig. 7e ). Furthermore, we found that the level of Spri-myc was decreased when strip was knocked down in S2 cells ( Fig. 7f , quantification in Fig. 7g), indicating that Strip affects the protein level of Spri. Together, these results suggest that Strip is involved in Spri-mediated Rab5 activation by stabilizing Spri. As Strip seems to regulate the activity of Rab5 by forming a complex with Spri, we examined whether a constitutively active form of Rab5 (Rab5CA, Rab5Q88L) could compensate for the loss of Strip function in early endosomes during axon elongation. Indeed, the strip dogi short-axon phenotype ( Fig. 7i ) was partially suppressed in strip dogi DL1 PN clones expressing Rab5CA ( Fig. 7j , quantification in Fig. 7l), with some axons even exhibiting L-shaped branching at the lateral horn ( Fig. 7j , white dotted circle). In contrast, the short-axon phenotype was enhanced in strip dogi DL1 PNs expressing a dominant-negative form of Rab5 (Rab5DN, Rab5S43N) ( Fig. 7k , quantification in Fig. 7l), that is, most of the axons were terminated at the calyx of the mushroom body ( Fig. 7l ‘class 3’). These data support our hypothesis that the Strip regulates axon elongation by controlling the activity of Rab5. During neural development, axon termini are exposed to a constantly changing surrounding environment. Thus, the spatio-temporal regulation of the amount of adhesion molecules and receptors at the axon growth cone is essential [6] . In this study, we identified uncharacterized protein Strip that forms complexes with Gl and Spri, and positively regulates clustering (retrograde transport along microtubule) of early endosomes. To form mature early endosomes from internalized small early endosomes, the coordination between clustering and fusion of early endosomes is crucial. For this, Strip serves as a molecular linker by interacting with Gl in clustering and with Spri, Rab5 and probably with Vps45 in fusion. Vps45 is a Sec-1/Munc18 (SM) protein that targets Avl to promote fusion of early endosomes, which seems to function with Strip in the wing development (genetic interactions among strip , Gl and regulators of early endosome fusion: Supplementary Fig. 6 ). As we also observed genetic interaction between spri and Gl in axon elongation ( Fig. 3l,o ), Strip seems to be a platform for early endosome organization by forming a dynein-Gl-Strip-Spri-Rab5 complex. Herein, we propose the following model to explain the physiological role of Strip in the organization of early endosomes ( Fig. 8 , See Fig. 8 legend for details). During axon elongation, the strength of the elongation signal could be properly regulated by the dynein-Gl-Strip-Spri-Rab5 complex by affecting the organization of mature early endosomes. Mature early endosomes are essential vesicular structures for cell signalling, serving both as signalling centres and as sorting centres to degrade or recycle cargoes. In vertebrate neurons, target-derived nerve growth factor (NGF) mediates axon elongation via retrograde axon transport of TrkA-containing signalling endosomes locally or to the cell body to stimulate the expression of downstream target genes essential for long-term axon growth and target innervation [7] , [8] . Furthermore, the amount of cell adhesion molecules might also be regulated by Strip-mediated early endosome organization. It has been reported that the regulation of the amount and localization of molecules such as L1 and integrin in the axon growth cone is essential for growth cone motility [9] . 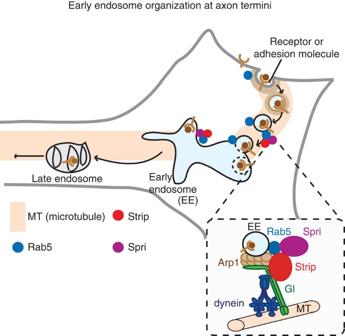Figure 8: Hypothetical model for the function of Strip in axon elongation. Strip (red) binds to the dynein accessory proteins Glued (green) and Spri (purple), and forms a complex with the Rab5 (blue)-containing early endosomes, suggesting that Strip seems to be in a large molecular complex, dynein-Gl-Strip-Spri-Rab5 complex (see the dotted rectangle). Thus, Strip seems to serve as a molecular linker of clustering and fusion steps of internalized small early endosomes, which is essential for the organization of mature early endosomes containing a ligand-receptor complex analogous to the vertebrate neurotrophin-TrkA complex that sends signals for axon growth. Figure 8: Hypothetical model for the function of Strip in axon elongation. Strip (red) binds to the dynein accessory proteins Glued (green) and Spri (purple), and forms a complex with the Rab5 (blue)-containing early endosomes, suggesting that Strip seems to be in a large molecular complex, dynein-Gl-Strip-Spri-Rab5 complex (see the dotted rectangle). Thus, Strip seems to serve as a molecular linker of clustering and fusion steps of internalized small early endosomes, which is essential for the organization of mature early endosomes containing a ligand-receptor complex analogous to the vertebrate neurotrophin-TrkA complex that sends signals for axon growth. Full size image Further investigations are still needed to identify which Strip domains are important for the formation of the dynein-Gl-Strip-Spri-Rab5 complex. As Gl and Spri were identified using a yeast two-hybrid screen, it seems that the binding between Gl and Strip, and that between Spri and Strip, are likely to be direct. Furthermore, we think that Gl and Spri bind to Strip simultaneously and form a tertiary complex for two reasons; (1) Spri and Gl showed genetic interaction in PNs and exhibited a phenotype similar to that of stip dogi PNs and (2) Vps45 and Gl exhibited genetic interaction at the wing vein formation ( Supplementary Fig. 6 ). Thus, Strip seems to serve as a molecular linker between early endosome clustering and fusion by simultaneously forming a complex with Gl and Spri. In addition, Strip seems to stabilize Spri protein level. Unfortunately, we were unable to produce a usable anti-Spri antibody; therefore, we could not examine Spri localization. However, we speculate that Spri stabilized by Strip could determine the spatio-temporal localization and the activity of Rab5. Regarding the binding between Strip and Gl, we hypothesize that Strip may act as an adaptor between early endosomes and dynein. Unlike the highly diverse kinesin superfamily proteins (KIFs), which encompass 45 genes, cytoplasmic dyneins have only two heavy-chain family members in mammals [3] . Thus, adaptor proteins for the dynein motor are thought to be important to determine the cargo selectivity, and some adaptor proteins have already been reported [3] , [50] , [51] . Although Kif16b links Rab5 and microtubules [52] , no specific molecule linking the dynein heavy chain with Rab5-positive early endosomes has been reported yet. Therefore, we speculate that Strip could serve as an adaptor protein between Rab5-positive early endosomes and the dynein/dynactin complex by binding to Gl, similar to RILP and ORP1L that serve as adaptors between late endosomes and the dynein/dynactin complex [50] , [51] . We have provided genetic evidences that Strip, Gl, Spri and Rab5 are required for both axon elongation and dendrite branching in PNs. However, the expression of a constitutively active form of Rab5 partially suppressed axon elongation and did not suppress dendrite branching defects of strip dogi PNs ( Fig. 7h–l , Supplementary Fig. 7 ). We consider that the level and the spatio-temporal pattern of Rab5 activity are crucial. Axon elongation and dendrite branching may require different levels or patterns of Rab5 activity. Furthermore, the failure to suppress the dendrite phenotype could also be explained by the fact that not only formation but also localization of mature early endosomes is required for dendrite branching. In Drosophila dendritic arborization (da) neurons, the proximal branching phenotype has been observed in the dendrite of Rab5 2 , dynein light intermediate chain ( dlic ) or the kinesin heavy chain ( khc ) mutant [20] . Consistent with this report, we also observed dendrite proximal branching phenotype in Rab5 2 or strip dogi PNs ( Figs 2e,f and 7a ). The additional dendrite branched out from the dendrite stalk at a more proximal side in Rab5 2 or strip dogi PNs than in wild-type PNs. Therefore, we hypothesized that the constitutively active form of Rab5 could not suppress the dendrite phenotype in strip dogi PNs, as the expression of the constitutively active form of Rab5 in strip dogi PNs could promote early endosome maturation in axon and dendrites, but could not adjust early endosome subcellular localization, which is crucial for dendrite branching. Strip is structurally and functionally conserved. Branching and elongation defects in strip dogi PNs were rescued by the expression of the mouse homologue, Strip1 ( Fig. 1f,j and n ). In addition, we also found that Strip1 is involved in neuronal migration in the mouse developing cerebral cortex ( Supplementary Fig. 8 ). In the mouse developing cerebral cortex, the Rab5-dependent endosomal trafficking pathway is required for neuronal migration [53] , rather than for neurite extension, probably because it occurs before dendrite formation and axon elongation in vivo . Electroporation of Strip1 shRNA into the cerebral cortex at E14 caused migration defects ( Supplementary Fig. 8 ), similar to those observed when Rab5 shRNAs were used [53] . Thus, strip/Strip1 is involved in Rab5-dependent neural development including neuronal morphogenesis and migration events in both Drosophila and the mouse. During our study of Strip function, Strip was reported as a member of the STRIPAK complex [23] , [24] , [42] . STRIPAK complex contains the PP2A phosphatase complex that is widely used as a phosphatase [22] . The core component of the PP2A phosphatase complex shows phosphatase activity, whereas the regulatory subunit determines the substrate specificity. Thus, PP2A phosphatase targets specific molecules by changing the regulatory subunit. When Strip is included in the PP2A complex, Cka serves as a regulatory subunit and targets Hippo and probably RAF that belongs to the RAS-MAPK pathway [23] , [24] . As early endosome organization is important for many signal-transduction pathways, it might be possible that axon elongation and dendrite targeting require both the dynein-Gl-Strip-Spri-Rab5 complex and the Strip-STRIPAK (Cka)-Hippo or the Strip-STRIPAK (Cka)-RAS-MAPK complex, but this does not seem possible, at least, in neuronal morphogenesis of PNs. When we generated PNs homozygous for Cka , we did not find any defects in axon elongation or dendrite branching ( Supplementary Fig. 9 ). Thus, we think that the Strip-STRIPAK complex might not have a major role in neuronal morphogenesis. The disruption of dynein or dynactin function causes neurodegeneration in many species, and this has been suggested to reflect impaired transport of signalling endosomes [54] . In humans, G59S and G59A missense mutations of p150 Glued have been discovered in motor neuropathy 7B [55] and Perry syndrome [56] , respectively. Both mutations are located within the p150 Glued cytoskeleton-associated protein glycine-rich (CAP-Gly) domain, which is an MT-binding domain required for efficient retrograde transport. Progressive motor neuron degeneration is observed in p150 Glued transgenic mice, with pathological similarities to amyotrophic lateral sclerosis (ALS), including muscle atrophy, axonal swelling, disrupted intracellular trafficking and proliferation of degenerative organelles such as lysosomes and autophagosomes [54] , [57] . Furthermore, motor neurons in Als2 (juvenile ALS-associated gene, Rab5GEF)-deficient mice show axonal degeneration. Moreover, the primary neurons in this mouse model show disturbed endosomal trafficking of the insulin-like growth factor 1 (IGF-1) and brain-derived neurotrophic factor (BDNF) receptors [54] . These observations suggest that retrograde transport and Rab5GEF may play a particularly important role in axonal health by transmitting information about the local environment from the axon to the soma. As Strip affects the early endosome organization by forming a complex with Gl and Spri, studying the functions of Strip may provide new insights into both developmental and pathological processes. Genetic mapping of strip dogi mutants The causal gene strip was mapped by single-nucleotide polymorphism (SNP)-based recombination [39] , which showed that the mutation responsible for the projection neuron (PN) phenotype in the strip dogi MARCM clone was at a cytological location between 63A and 64A. Next, assuming that strip dogi is homozygous lethal, we performed a lethal complementation test with deficiency lines available for this candidate region. Df(3L)HR232 and Df(3L)HR119 failed to complement the strip dogi lethality, suggesting that the strip dogi chromosome maps within the genomic region from 63C02 to 63D02 (~130 kb). We next measured the recombination rate from genetically mapped P-element insertion sites [40] . While generating recombinant lines, we obtained three independent recombinants that complemented the strip dogi lethality; analysis of their recombination points narrowed the candidate region down to ~28 kb. Next, we generated a small deficiency, Df(tc-1) (~7 kb) ( Fig. 1o ), using the f05249 and e04482 PiggyBac lines. Df(tc-1) failed to complement the strip dogi lethality. Furthermore, we made shRNA-strip and PNs expressing shRNA-strip exhibited the phenotypes similar to those observed in strip dogi PN clones ( Supplementary Fig. 1d–f ). In addition, Strip protein expression was significantly reduced in strip dogi homozygous embryos ( Fig. 1p ). Lastly, we confirmed that UAS-strip could mostly rescue the strip dogi PN clone phenotypes ( Fig. 1e,i,m ), indicating that strip was the gene responsible for these phenotypes. Clonal analysis We used the MARCM method [58] . In brief, we crossed MARCM ready flies that contain FLP recombinase, an FRT site, GAL4 , tubulin 1 promoter- GAL80 and UAS-mCD8GFP/RFP to a line containing the corresponding FRT and mutation of interest for MARCM analysis. To induce MARCM neuroblast clones, we heat-shocked (37 °C, 1 h) flies with the appropriate genotype for 0–24 h after larval hatching (ALH). To analyse DL1 PNs, we heat-shocked flies (37 °C, 1 h) with the appropriate genotypes at 0–30 h ALH for Fig. 1g,h,k, and l or at 0–24 h ALH for other analyses. The anterodorsal PN single-cell clones generated in this time period innervate the DL1 glomerulus. Dissections were performed on both genders of adults aged 1–10 days, with the exception of those described in Fig. 4a–f (21 h after puparium formation, APF) and Supplementary Fig. 1m–o (0 h APF). Fly strains The genotypes of Drosophila melanogaster used in each experiment are shown in Supplementary Table 1 . Flies were maintained under standard laboratory condition (25 °C). Both genders of adults aged 1–10 days are used for most studies. As for Supplementary Figs 2a–d and 6 , adults aged 1–2 days were used. Gl 1 , UAS-YFP-Rab5 (ref. 49 ) , UAS-YFP-Rab5S43N [49] , UAS-YFP-Rab5Q88L [49] , and daughterless (da)-Gal4 were obtained from the Bloomington Stock Centre. Rab5 2 and UAS-GFP-myc-2 x FYVE were kind gifts from Marcos González-Gaitán [47] , UAS-syt-HA is a kind gift from Thomas Schwarz [46] , UAS-Vps45-RNAi , Vps45 JJ2 and avl 1 were kind gifts from David Bilder [15] , [48] , [59] and Cka 1 is a kind gift from Steven X. Hou [60] . DNA construction and generation of transgenic flies To generate UAS-strip , UAS-strip-V5 and UAS-FLAG-strip flies, strip cDNA was amplified by PCR using the EST clone (AT25231) and was subcloned into pUAST . A V5 epitope tag was added at the strip C terminus or a FLAG epitope tag was added at the strip N terminus. The cDNA of Mus musculus Strip1 was amplified by PCR using the BC023952 EST clone. As the 12 bp of N-terminal sequence of this clone is reported not to align with the mouse genome, we corrected the sequence and subcloned it into pUAST . Transgenic flies were generated by BestGene Inc. The generation of shRNA-strip , shRNA-Gl , shRNA-sprint and UAS-resistant-strip was designed as follows [61] . The two sites targeted by shRNA-strip were shRNA-strip-6 : 5′- ATGGCTTGGAAACAGAAAAATA -3′ and shRNA-strip-9 : 5′- CGGCCACAGCTACTGATATACT -3′; the two sites targeted by shRNA-Gl were shRNA-Gl-1 : 5′- GCGAACTAATACCGGTATTATC -3′ and shRNA-Gl-7 : 5′- GGACCGACACAGAACTTTAAGA -3′; the two sites targeted by shRNA-spri were shRNA-sprint-2 : 5′- TTCAGCGGATTACTCATTAAGA -3′ and shRNA-sprint-10 : 5′- GCGGCCAGTAATCCCTTTAATG -3′. For UAS-resistant-strip , the twentieth nucleotide of the strip-shRNA-9 target site was altered from A to T. These shRNAs were subcloned into pUAST or pUASTattB , and transgenic flies were generated by BestGene Inc. To generate UAS-spri-myc , sprint cDNA was amplified by PCR using the EST clone (SD06366) and was subcloned in pUAST . A c-myc epitope tag was added at the C terminus of sprint . To generate shRNA-Strip1 , we used the Whitehead Institute’s siRNA prediction tool to research target sites ( http://sirna.wi.mit.edu/ ). We inserted oligonucleotides targeting four distinct regions in the Strip1 -coding sequence ( shRNA-Strip1-1 : 5′- GAATTCCTGATGAATCGAA -3′, shRNA-Strip1-2 : 5′- CTATAAGGCTGACGACTCT -3′, shRNA-Strip1-3 : 5′- GTTGAACCACATCTACCAG -3′, shRNA-Strip1-4 : 5′- CGTACGGCAATGATCTTGA -3′) into the pSilencer 3.0-H1 neo vector (Ambion). All of these regions contained a hairpin loop sequence (5′- TTCAAGAGA -3′). To generate pcDNA3-Strip1-V5 , we added a V5 epitope tag to the C terminus of Strip1 cDNA and subcloned it into pcDNA3 . Detailed DNA constructions are available upon request. Bioinformatics For homology searches, we used the InParanoid: Eukaryotic Ortholog Groups ( http://inparanoid.sbc.su.se/cgi-bin/index.cgi ). Identity and similarity were calculated by the GENETYX-MAC. ClustalW ( http://clustalw.ddbj.nig.ac.jp/top-j.html ) was used to generate a phylogenetic tree of the strip homologs ( Supplementary Fig. 1k ). Anti-Strip antibody generation We generated a recombinant protein representing a 91-amino-acid hydrophilic region of Drosophila Strip (amino acid 309 to 399 of PB, 264 to 354 of PA) in E. coli ( pCold vector). The recombinant protein was purified and injected into rabbits or rats to generate polyclonal or monoclonal antibodies, respectively. The IgG fraction of the polyclonal antibody was purified. Antibody generation was performed by the Hokudo Co., Ltd. Immunohistochemistry The fixation and immunostaining of fly brains were carried out as follows [62] . Brains were dissected in 0.3% Triton X-100 (vol/vol) in phosphate-buffer (PBT), followed by fixing in 4% paraformaldehyde (PFA) (wt/vol) with 0.3% Triton X-100 (vol/vol) in PBT at RT for 20 min, and subsequently blocked in PBT with 5% normal goat serum (vol/vol) for 1 h at RT. Primary and secondary antibody incubation were carried out in PBST for overnight at 4 °C. For Fig. 4a–f , pupal brains were dissected in cold Schneider’s medium and incubated with primary antibody in Schneider’s medium with 10% normal goat serum (vol/vol) at RT for 1 h, followed by quickly rinsing with cold PBS for 3 times and fixing in 4% PFA (vol/vol) in PBS at RT for 20 min. Subsequent blocking and antibody incubation were similar with adult brains. For Drosophila S2 cells, cells were cultured on Concanavalin A-coated coverslips, fixed, and immunostained as follows [62] . S2 cells were grown for 1 h at 26 °C on Concanavalin A-coated coverslips, and were fixed for 20 min in 4% PFA (wt/vol) with 0.3% Triton X-100 (vol/vol) in phosphate-buffer saline (PBST) at RT for 10 min, and subsequently blocked in PBST with 5% normal goat serum (vol/vol) for 30 min. Primary and secondary antibody incubation were carried out in blocking solution for 1 h at RT. For HeLa cells, cells were cultured on polyethylene-imine-coated cover slips, fixed, and immunostained as with the S2 cells. We used the following antibodies: nc82 (mouse, 1:40, DSHB), the anti-mCD8 (rat, 1:200, Invitrogen), anti-GFP (mouse, 1:1,000, Clontech), the anti-DsRed (rabbit, 1:500, Clontech), anti-HA 12CA5 (mouse, 0.8 μg/ml, Roche), and anti-EEA1 (mouse, 1:500, BD Transduction Laboratories) antibodies. The anti-Rab5 (ref. 47 ) (rabbit, 1:1,000) and the anti-Avl [48] (rabbit, 1:200) antibodies are kind gifts from Marcos González-Gaitán, David Bilder and Thomas Vaccari. The anti-Strip (rat) was generated as described above (1:50). Immunoprecipitation and immunoblotting S2 cell were sonicated in lysis buffer (25 mM Tris-HCl, pH 7.9, 10 mM NaCl, 2 mM EDTA, 0.5% Triton X-100, 10 mM DTT, and 1 × cOmplete (cocktail of protease inhibitors, Roche)) and incubated with anti-Strip antibody (rat, 1:100) or control IgG overnight. Protein G agarose (Roche) was added, and immunoprecipitation was performed according to the manufacturer’s protocol. For the immunoprecipitation of c-myc tagged Sprint, S2 cells transfected with Actin-Gal4 (pAcPa-Actin5c-Gal4) , UAS-spri-myc and UAS-FLAG-strip were lysed and incubated with EZview Red Anti-c-Myc Affinity Gel (Sigma). For the immunoprecipitation of YFP tagged Rab5, Rab5WT, Rab5CA, and Rab5DN were subcloned in pUAST at first; Rab5WT, Rab5CA, and Rab5DN were amplified by PCR using UAS-YFP-Rab5WT [49] , UAS-YFP-Rab5Q88L [49] , and UAS-YRP-Rab5S43N [49] flies as template. S2 cells transfected with Actin-Gal4 , UAS-spri-myc and UAS-YFP-Rab5 WT/CA/DN were lysed and incubated with anti-GFP antibody (rabbit, 1:500, MBL) overnight. Protein G agarose (Roche) was added and immunoprecipitation was performed according to the manufacturer’s protocol. Western blotting was performed according to standard techniques. Briefly, we subjected 2–10 μg of S2 cell lysates or embryo lysates to SDS-PAGE analysis (12.5% for Histon H3 and Rab5 detection; for others, 7.5 or 10%) and immunoblotting. The following antibodies were used for immunoblotting: the anti-Strip antibody (rabbit, 1:200), the anti-Strip antibody (rat, 1:50), the anti-α-tubulin (mouse, 1:2,000, Sigma), the anti-Gl C-term antibody [27] (rabbit, 1:2,000), the anti-GFP antibody (mouse, 1:2,000, Roche), anti-myc antibody (mouse, 1:1,000, Invitrogen), anti-FLAG antibody (mouse, 1:1,000, Sigma), anti-V5 antibody (mouse, 1:200, Invitrogen), anti-GST (mouse, 1:200, Santa Cruz Biotechnology), and the anti-Histone H3 antibody (rabbit, 1:2,000, Active motif). The anti-Rab5 antibody [47] (rabbit, 1:1,000) is a kind gift from M. González-Gaitán. All data are representative of more than three biological replicates. Images of the full blots for all western blots are provided in Supplementary Fig. 10 . GST pull-down The Gl fragment from 676 to 914 amino acids was amplified from genomic DNA and the Spri fragment from 1,404 to1,700 amino acids were amplified by PCR using EST clone (SD06366). Both of these fragments were subcloned into pGEX-5X3 . GST, GST-Gl (676–914 a.a.), or GST-Spri (1,404–1,700 a.a.) was expressed in BL21 (DE3) bacterial cells and purified with Glutathione Sepharose 4 Fast Flow (GE). These glutathione sepharose beads were co-incubated with embryo lysates ( UAS-strip-V5/+; daughterless (da)-Gal4/+ or da-Gal4/ UAS-FLAG-strip ) collected at 0–22 h after egg laying. Yeast two-hybrid screening For yeast two-hybrid screening, the full length of strip was used as bait and the Drosophila whole-embryo library was used as prey; the screening was performed by the Hybrigenics. dsRNA generation and treatment The dsRNA design, production, and treatment were performed as follows [63] . 700–900 bp gene-specific sequences with T7 RNA polymerase sequence at both ends were amplified by PCR and in vitro transcription was performed using T7 RiboMAX Express RNAi System (Promega) according to the manufacturer’s protocol. For strip dsRNA, templates for in vitro transcription were generated using the primers 5′- TAATACGACTCACTATAGGGCCTGCATAAACCTGCTGCGC -3′ and 5′- TAATACGACTCACTATAGGGCTAGAGGGCGTCCCAGTCGG -3′. For control and Gl dsRNA, primer sequences were used to amplify the sequence from the bacterial cloning plasmid pBluescript SK [63] and the Gl C-terminus [27] . Cells (1.0 × 10 6 ) were cultured in a 35-mm dish; 30 μg dsRNA was applied every two days until the cells were used for analysis. For Fig. 5 , cells were treated with control, strip , or Gl dsRNA for 8 days. For Fig. 7f , S2 cells that stably express YFP-Rab5 were transfected with Actin-Gal4 and UAS-sprint-myc for two days and split into half to treat with control or strip dsRNA for 6 days. Transfection with shRNA Actin-Gal4 and desired UAS construct ( UAS-shRNA-strip, UAS-FLAG-strip, UAS-spri-myc, UAS-YFP-Rab5WT, DN, or CA ) were co-transfected using Effectene Transfection Reagent (Qiagen); 2.0 × 10 6 Drosophila S2 cells for 35-mm dish, 6.0 × 10 6 cells for 60-mm dish were plated and transfection was performed according to the manufacturer’s protocol. Cells were collected for immunoblots 48 h after transfection. pcDNA3-Strip1-V5 and shRNA-Strip1-1, 2, 3 or 4 were co-transfected using Lipofectamin 2,000 (Invitrogen); 1.0 × 10 5 HEK293T cells were plated on a 35-mm dish, and transfection was performed according to the manufacturer’s protocol. Cells were collected for immunoblots 24 h after transfection. FM1-43 dye assay Drosophila S2 cells were plated on Concanavalin A-coated cover slips, and treated with 5 μg/ml FM1-43 dye (Molecular Probes)/ HBSS for 1 min, and incubated for 5 min at 25 °C after a quick wash, and fixed immediately with 4% (vol/vol) PFA/HBSS without washing. Fixation was 10 min at RT. Cells were mounted with SlowFade® Gold antifade reagent with DAPI (Invitrogen). EGF-Alexa488 uptake assay in HeLa cells Dharmacon siGENOME non-Targeting siRNA Pool #1 (D-00126-13-05) (100 nM) or siGENOME SMARTpoll human STRIP1 (M-02516091-005) (100 nM) was transfected into HeLa cells (1.0 × 10 5 ) with Lipofectamin 2,000 (Invitrogen) according to manufacturer’s protocol, cultured for 3 days, and plated on polyethylene-imine-coated cover slips for over night. Cells were pulsed with Alexa Fluor 488 EGF complex (Invitrogen) for 3 min and immediately fixed or rinsed and incubated for 27 min at 37 °C and fixed. Electroporation in utero Animals were handled according to the guidelines established by the University of Tokyo and Keio University. All the electroporations were performed on E14 embryos. Electroporation in utero and the measurement of EGFP fluorescence intensity in various regions of the cerebral cortex were performed as follows [53] . Fluorescent images of frozen section of EGFP expressing mouse brains were captured by TCS-SP5 laser scanning confocal microscopy (Leica). Fluorescence intensities inside similar width rectangles in various regions of the cerebral cortex (layers II–IV, V–VI, IZ, and SVZ/VZ) were measured by the Leica SP5 software. Relative intensities to the total fluorescence were calculated and plotted in the graphs with standard errors. Image acquisition For all experiments other than HeLa cell imaging, images were obtained using TCS-SP5 laser scanning confocal microscopy (Leica) with a PL APO CS 40x/1.25 Oil lens (Leica) for PN imaging or a PL APO CS 63x/1.40 Oil lens (Leica) for imaging of S2 cells. For imaging of HeLa cells, TCS-SP8 laser scanning confocal microscopy (Leica) with a PL APO CS 63x/1.40 Oil lens was used. Fields of view were randomly selected and all experiments were repeated more than three times. For PN clones other than Fig. 4 , more than 10 clones were imaged and representative images were shown in Figures. For PN clones of Fig. 4 , S2 cells and HeLa cells, the exact number of samples imaged was shown in each Figure. Image analysis For Fig. 4 , fluorescence intensities of FYVE-GFP and mCD8RFP inside axon stalks (200 μm 2 ) were measured by the Leica SP5 software. For Fig. 5 , image analysis was performed using the Particle Analyzer of ImageJ software. Single section that passes the centre of cells was selected for each S2 cell stained with the anti-Rab5 antibody or the anti-Avl antibody, and the size of vesicles was determined by using the particle analyzer. For Fig. 6 , Fig. 7l , and Supplementary Fig. 2k , all images were blinded prior to the classification to avoid experimental bias. The investigator who conducted the blind test was totally independent from the investigator who performed experiments. Statistical analysis Statistical analysis was performed using Prism software (GraphPad). Unpaired two-tailed t -tests were used to compare the GFP-FYVE intensity between control and strip PNs, and for the quantitative analysis of the extent of cell migration in the mice cerebral cortex. The chi-square test was used to compare data variations among control, strip , or Gl dsRNA-treated S2 cells or between control and STRIP1 siRNA-treated HeLa cells. The chi-squre test was also used to compare data variations of synaptotagmin localization between control or strip dogi PNs. Exact P -values are provided unless P <0.0001. How to cite this article : Sakuma, C. et al . Drosophila Strip serves as a platform for early endosome organization during axon elongation. Nat. Commun. 5:5180 doi: 10.1038/ncomms6180 (2014).